Phosphorylation of LRRK2 by casein kinase 1α regulatestrans-Golgi clustering via differential interaction with ARHGEF7 LRRK2, a gene relevant to Parkinson's disease, encodes a scaffolding protein with both GTPase and kinase activities. LRRK2 protein is itself phosphorylated and therefore is subject to regulation by cell signalling; however, the kinase(s) responsible for this event have not been definitively identified. Here using an unbiased siRNA kinome screen, we identify and validate casein kinase 1α (CK1α) as being responsible for LRRK2 phosphorylation, including in the adult mouse striatum. We further show that LRRK2 recruitment to TGN46-positive Golgi-derived vesicles is modulated by constitutive LRRK2 phosphorylation by CK1α. These effects are mediated by differential protein interactions of LRRK2 with a guanine nucleotide exchange factor, ARHGEF7. These pathways are therefore likely involved in the physiological maintenance of the Golgi in cells, which may play a role in the pathogenesis of Parkinson’s disease. Genetic variations in Leucine-rich repeat kinase 2 ( LRRK2 ) are linked to both familial and sporadic Parkinson’s disease (PD) [1] . LRRK2 is a large multidomain protein of 2,527 amino acids and is made up of an enzymatic core (ROC (Ras of complex)–COR (C-terminal of ROC)-kinase) and nonenzymatic domains (ankyrin, LRR and WD40) ( Fig. 1a ) [2] . Pathogenic mutations are clustered in the enzymatic regions and cause either a decrease in GTPase activity or an increase in kinase activity [3] , [4] , [5] , [6] , [7] . These results suggest that altered activity of LRRK2 is important for pathogenesis of PD and might represent a therapeutic target, although the mechanism(s) involved remain unclear as no unambiguous kinase substrate(s) for LRRK2 have been identified. 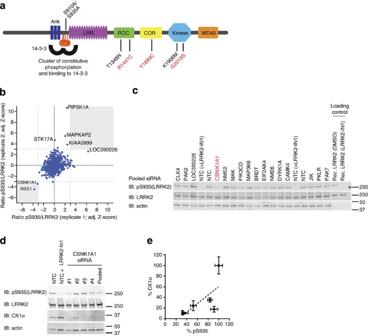Figure 1: Casein kinase 1 alpha is a kinase regulator of LRRK2. (a) Schematic of the domain organization and location of LRRK2 constitutive phosphorylation sites. Domains include ankyrin (Ank), leucine-rich-repeat (LRR), ROC proteins, COR, kinase and WD40 domains. Constitutive phosphorylation sites are clustered upstream of the LRR domain and are crucial for binding to 14-3-3 proteins. Pathogenic mutations, shown in red (R1441C, Y1699C and G2019S; N1437S not shown), S910A/S935A, T1348N and K1906M, shown in black, are designed mutants used to block 14-3-3 binding, GTP/GDP binding and kinase activity, respectively. (b) RNAi screen against kinases to identify kinase regulators of LRRK2 at S935. The screen was performed in duplicate per siRNA pool and each value of ratio pS935/LRRK2 was converted with a Z-transformation, adjusted for date of assay. Hits were identified if both replicates were 3 s.d. Z away from the mean.CSNK1A1andWEE1were two candidates with adjusted Z<−3.0 in both duplicates (bottom left grey box). (c) Western blot example from the RNAi screen identifyingCSNK1A1as the candidate kinase for S935 LRRK2. Recombinant LRRK2, purified from cells pretreated with DMSO or LRRK2-IN1, were included in each blot as loading control to allow for normalization across blots. (d)CSNK1A1validated using single siRNAs and pooled siRNAs. Three of four singleCSNK1A1siRNAs showed that when CK1α was knocked down, S935 phosphorylation was also reduced. Representative blots from three independent experiments. NTC, nontargeting control, singleCSNK1A1siRNAs no.1, 2, 3, 4 (used at 6.25 nM final concentration). (e) Quantitation of blots ind. Graph shows the mean±s.e.m. (n=3) for relative CK1α and phosphorylated LRRK2 signals. Figure 1: Casein kinase 1 alpha is a kinase regulator of LRRK2. ( a ) Schematic of the domain organization and location of LRRK2 constitutive phosphorylation sites. Domains include ankyrin (Ank), leucine-rich-repeat (LRR), ROC proteins, COR, kinase and WD40 domains. Constitutive phosphorylation sites are clustered upstream of the LRR domain and are crucial for binding to 14-3-3 proteins. Pathogenic mutations, shown in red (R1441C, Y1699C and G2019S; N1437S not shown), S910A/S935A, T1348N and K1906M, shown in black, are designed mutants used to block 14-3-3 binding, GTP/GDP binding and kinase activity, respectively. ( b ) RNAi screen against kinases to identify kinase regulators of LRRK2 at S935. The screen was performed in duplicate per siRNA pool and each value of ratio pS935/LRRK2 was converted with a Z-transformation, adjusted for date of assay. Hits were identified if both replicates were 3 s.d. Z away from the mean. CSNK1A1 and WEE1 were two candidates with adjusted Z<−3.0 in both duplicates (bottom left grey box). ( c ) Western blot example from the RNAi screen identifying CSNK1A1 as the candidate kinase for S935 LRRK2. Recombinant LRRK2, purified from cells pretreated with DMSO or LRRK2-IN1, were included in each blot as loading control to allow for normalization across blots. ( d ) CSNK1A1 validated using single siRNAs and pooled siRNAs. Three of four single CSNK1A1 siRNAs showed that when CK1α was knocked down, S935 phosphorylation was also reduced. Representative blots from three independent experiments. NTC, nontargeting control, single CSNK1A1 siRNAs no.1, 2, 3, 4 (used at 6.25 nM final concentration). ( e ) Quantitation of blots in d . Graph shows the mean±s.e.m. ( n =3) for relative CK1α and phosphorylated LRRK2 signals. Full size image However, LRRK2 is itself subject to regulation by cellular signalling pathways. LRRK2 is constitutively phosphorylated at multiple sites in a region N terminal to the LRR domain including serines 910 and 935 (refs 8 , 9 , 10 , 11 ). Phosphorylation of these sites is crucial in maintaining binding to 14-3-3 proteins. These sites are phosphorylated on kinase dead LRRK2 and therefore must come from another, as yet unidentified, kinase. However, acute inhibition of LRRK2 kinase activity causes diminished LRRK2 phosphorylation and 14-3-3 interaction, accompanied by redistribution of LRRK2 into discrete cytoplasmic structures [9] , [12] , [13] , [14] , [15] , [16] . Several pathogenic PD mutations, including those in the ROC-COR domain that diminish GTPase activity, have diminished S910/S935 phosphorylation, lower 14-3-3 binding and formation of inclusions [9] , [17] . Collectively, these observations show that there is feedback regulation between constitutive phosphorylation and LRRK2 activity and suggest that the GTP-binding capacity of LRRK2 is important in this process. Understanding the nature of LRRK2 regulation may be critical for developing novel therapeutic approaches for PD. Specifically, it has been proposed that kinase inhibitors are therapeutically useful, but the literature discussed above show that this also changes LRRK2 signalling and may therefore have pleiotropic effects on the cell. Here we set out to identify the kinase(s) that are responsible for LRRK2 phosphorylation and, from there, to dissect out the relative effects of kinase inhibition compared with loss of constitutive phosphorylation. Using short interfering RNA (siRNA) and pharmacological approaches, we identified casein kinase 1 alpha (CK1α) as a kinase responsible for LRRK2 phosphorylation at S910/S935. We show that there is a relationship between constitutive phosphorylation and Rab7L1-dependent Golgi clustering [18] , [19] that is mediated, at least in part, by the interacting protein ARHGEF7. We therefore propose that LRRK2 phosphorylation and kinase activity are important and distinct regulatory events for the overall function of LRRK2 leading to altered downstream signalling events, in particular the maintenance of Golgi in cells, which could play a role in the pathogenesis of LRRK2-PD. CK1α phosphorylates LRRK2 at S910 and S935 To identify the kinase(s) responsible for the constitutive phosphorylation of LRRK2, we performed a kinome-wide siRNA screen. To generate a positive control for dephosphorylation, we started by replicating previous data on the LRRK2 inhibitor LRRK2-IN1 (ref. 12 ). Treatment of stable HEK293T cell lines expressing FLAG-tagged LRRK2 variants with 1 μM LRRK2-IN1 for 2 h (h) caused loss of constitutive phosphorylation ( Supplementary Fig. 1a,b ), accompanied by loss of binding of 14-3-3 proteins ( Supplementary Fig. 1b,c ). Interestingly, the S910A/935A mutation in LRRK2, where two known phosphorylation sites are unavailable, was still radiolabelled ( Supplementary Fig. 1a ), demonstrating that LRRK2 is phosphorylated at additional sites and that the S910A/S935A mutation is not a full mimic of complete dephosphorylation. Hsp90 binding was retained under conditions of LRRK2 inhibition, showing that phosphorylation controls interaction with subsets of LRRK2-binding partners ( Supplementary Fig. 1c ). Moreover in agreement with previous results [17] , mutations in LRRK2 including R1441C in the ROC domain and Y1699C in the COR domain were not basally phosphorylated and did not bind 14-3-3 ( Supplementary Fig. 1b,c ). The pathogenic G2019S mutation in the kinase domain is phosphorylated and sensitive to the effects of LRRK2-IN1, whereas the artificial kinase dead mutation K1906M is phosphorylated but resistant to LRRK2-IN1. These results confirm that acute kinase inhibition causes a loss of phosphorylation of LRRK2 in a manner that is dependent on LRRK2 kinase activity itself, as previously reported. We next developed a high-throughput assay with stable HEK293T cell lines expressing FLAG-tagged wild-type (WT) LRRK2 (refs 20 , 21 ). We screened siRNAs against ~700 kinases in duplicate for their ability to alter the phosphorylation of S935 of LRRK2. Cells treated with LRRK2-IN1 were used on each plate as a positive control to confirm assay performance. After normalization, we identified candidate kinases using the criteria that the adjusted Z -score for the ratio of pS935/total LRRK2 was −3 or greater, that is, was more than three s.d.’s below the mean ( Fig. 1b,c ). This gave us two candidate kinases; CK1α ( CSNK1A1 , Z=−3.14, −3.44) and WEE1 ( WEE1 , Z=−3.73, −4.45). Given that WEE1 is largely nuclear [22] and CK1α is cytoplasmic and has a similar cellular distribution to LRRK2, we focused on CK1α. The kinome library used in the screen contained multiple pooled independent siRNA constructs per gene. To validate the initial results, we tested each of the four independent CSNK1A1 siRNA sequences for their ability to induce dephosphorylation of LRRK2 at S935 ( Fig. 1d ). There was a positive correlation between the relative amount of CK1α protein and the relative degree of LRRK2 phosphorylation ( Fig. 1e ). We further validated CK1α as a candidate kinase for LRRK2 using a pharmacological approach. Two structurally distinct CK1 inhibitors, IC261 and D4476, inhibited LRRK2 phosphorylation at S935 ( Fig. 2a ) and S910 ( Supplementary Fig. 2 ). However, the CK2 inhibitor 4,5-dihydro-N-(2,3,5,6-tetrabromo-4-methoxyphenyl)-1H-imidazole-2-carboxamide (TMCB) had no effect ( Fig. 2a ). In the same experiments, we also examined the kinase dead LRRK2 mutant K1906M. In contrast to LRRK2-IN1, CK1 inhibitors were able to cause the dephosphorylation of both WT and K1906M LRRK2 ( Fig. 2a ). Titration of the most effective inhibitor, IC261, showed that the effects were quantitatively comparable for both WT and K1906M, with an estimated IC50 of 176 and 152 μM, respectively ( Fig. 2b ). We also tested whether the amount of dephosphorylation of LRRK2 after treatment with CK1 inhibitors was sufficient to induce loss of 14-3-3 binding. Consistent with the experiments above, we found loss of pS935 immunoreactivity and a concomitant decrease in 14-3-3 binding after treatment with IC261 ( Fig. 2c,d ). 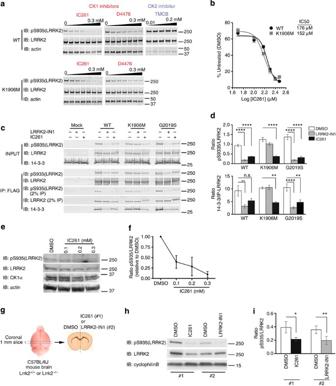Figure 2: Pharmacological inhibition of CK1α results in loss of pS935 and 14-3-3 binding. (a) Inhibition of with CK1, but not CK2, specific kinase inhibitors causes dephosphorylation of pS935 of WT and K1906M in a dose-dependent manner. Representative blots of three independent experiments. (b) Dose response curve of IC261 on phosphorylation of S935 quantified from 2a. IC50 for WT=~176 μM, IC50 for K1906M=152 μM. Graph shows mean±s.e.m. (n=3). (c) CK1α inhibition with 200 μM IC261 abolishes LRRK2/14-3-3 interaction. Representative blots from four independent experiments. (d) Quantitation of blots inc. Graph shows mean±s.e.m. (n=3). Statistical significance tested with two-way ANOVA with Bonferronipost hoctest (**P<0.01; ****P<0.0001). (e) CK1α inhibition with IC261 in 14 DIV neurons showed a dose-dependent decrease of endogenous pS935. Representative blots from three independent experiments. (f) Quantitation of blots ine. Graph shows mean±s.e.m. (g) Experimental overview of acute brainex vivoexperiment. Coronal brain slices of 1-mm thickness were prepared, and slices from one half of the brain from the same animal were treated with DMSO and the other half with either IC261 (no.1) or LRRK2-IN1 (no.2). (h) Adult nontransgenic WT mouse (4–9 weeks) acute brainex vivoslices treated with DMSO, 1 μM LRRK2-IN1 and 300 μM IC261 for 2 h. S935 phosphorylation was reduced upon treatment with LRRK2-IN1 and IC261. (i) Quantitation of blots in 2 h. Graph shows mean±s.e.m. (n=7). Statistical significance tested with pairedt-test comparing treatments within a group (*P<0.05; **P<0.01). Figure 2: Pharmacological inhibition of CK1α results in loss of pS935 and 14-3-3 binding. ( a ) Inhibition of with CK1, but not CK2, specific kinase inhibitors causes dephosphorylation of pS935 of WT and K1906M in a dose-dependent manner. Representative blots of three independent experiments. ( b ) Dose response curve of IC261 on phosphorylation of S935 quantified from 2a. IC50 for WT=~176 μM, IC50 for K1906M=152 μM. Graph shows mean±s.e.m. ( n =3). ( c ) CK1α inhibition with 200 μM IC261 abolishes LRRK2/14-3-3 interaction. Representative blots from four independent experiments. ( d ) Quantitation of blots in c . Graph shows mean±s.e.m. ( n =3). Statistical significance tested with two-way ANOVA with Bonferroni post hoc test (** P <0.01; **** P <0.0001). ( e ) CK1α inhibition with IC261 in 14 DIV neurons showed a dose-dependent decrease of endogenous pS935. Representative blots from three independent experiments. ( f ) Quantitation of blots in e . Graph shows mean±s.e.m. ( g ) Experimental overview of acute brain ex vivo experiment. Coronal brain slices of 1-mm thickness were prepared, and slices from one half of the brain from the same animal were treated with DMSO and the other half with either IC261 (no.1) or LRRK2-IN1 (no.2). ( h ) Adult nontransgenic WT mouse (4–9 weeks) acute brain ex vivo slices treated with DMSO, 1 μM LRRK2-IN1 and 300 μM IC261 for 2 h. S935 phosphorylation was reduced upon treatment with LRRK2-IN1 and IC261. ( i ) Quantitation of blots in 2 h. Graph shows mean±s.e.m. ( n =7). Statistical significance tested with paired t -test comparing treatments within a group (* P <0.05; ** P <0.01). Full size image To ensure that our results in HEK293FT cells were relevant to LRRK2 biology in neurons and at endogenous levels, we treated nontransgenic WT mouse primary cortical neuron cultures ( Fig. 2e,f ) and acute adult brain slices ( Fig. 2g–i ) with IC261 and measured pS935 levels. We first performed a dose-dependent assay using cultured neurons and showed that endogenous LRRK2 in cultured neurons was dephosphorylated at S935 with increasing IC261 concentrations ( Fig. 2e,f ). We were also able to demonstrate a similar loss of S935 phosphorylation upon IC261 and LRRK2-IN1 treatment in acute brain slices from adult mice ( Fig. 2g–i ). CK1α is expressed in both primary cultured neurons ( Fig. 2e ) and in the adult brain ( Supplementary Fig. 3b ). To verify that the proteins detected were specific to phosho- and total LRRK2, we included primary neuronal cultures and acute brain slices from LRRK2 knockout mice ( Supplementary Fig. 3a,b ). Taken together, our in vitro and ex vivo results support that CK1α is a physiologically relevant kinase for LRRK2 phosphorylation in the brain. CK1α directly phosphorylates LRRK2 The combined siRNA and pharmacological data suggest that CK1α influences the phosphorylation of LRRK2 but does not address whether CK1α directly acts on S935 or plays an upstream, regulatory role. To determine whether LRRK2 is a direct substrate of CK1α, we incubated purified LRRK2 with recombinant CK1α in kinase buffer in vitro . Recombinant CK1α could phosphorylate LRRK2, without any additional components, not only at S910 and S935, but also at S955 and S973 ( Fig. 3a ). Sequence analysis ( Fig. 3b ) shows that these serines are in a weak consensus site for CK1α. Addition of IC261 prevented the increase in S935 signal but the LRRK2 inhibitor, LRRK2-IN1, did not as expected ( Fig. 3c,d ). These results suggest that, although LRRK2-IN1 inhibits other kinases [23] , CK1α is not one of them, which we confirmed by incubating recombinant CK1α with LRRK2-IN1 in vitro ( Supplementary Fig. 4a,b ). 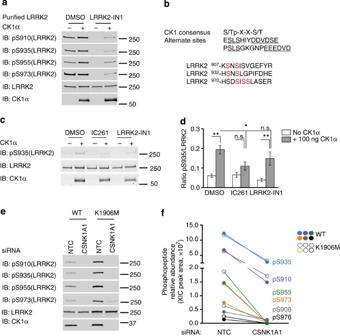Figure 3: CK1α directly phosphorylates LRRK2in vitroandin vivo. (a) LRRK2 is a substrate of CK1α. CK1α phosphorylates LRRK2,in vitro, at S910, S935, S955 and S973 sites. Representative blots of three independent experiments. (b) Consensus sequence of CK1 phosphorylation. The S/Tp-X-X-S/T is the canonical phosphorylation motif42. Alternative phosphorylation motif of CK1 consists of an SLS motif followed by an acidic cluster in positionsn+7 (underlined43). Sequence analysis of LRRK2 shows that serines 910, 935 and other constitutively phosphorylated serines at 973/975/976 is a weak consensus site for canonical and noncanonical CK1α phosphorylation. Phosphorylated serines of LRRK2 are shown in red. (c) IC261, but not LRRK2-IN1, inhibited CK1α phosphorylation of LRRK2in vitro. Concentrations of inhibitors used were 50 μM IC261 and 100 nM LRRK2-IN1. Results were consistent even when higher concentration of inhibitor, 100 μM IC261 and 1 μM LRRK2-IN1, was used (Supplementary Fig. 4b). Representative blots of three independent experiments. (d) Quantitation of blots inc. Graph shows mean±s.e.m. Statistical significance tested with two-way ANOVA with Bonferronipost hoctest (*P<0.05; **P<0.01; n.s.=not significant). (e) LRRK2 is dephosphorylated at S910, S935, S955 and S973 upon knockdown withCSNK1A1siRNA in a LRRK2-kinase-independent manner, as both WT and K1906M is dephosphorylated to the same extent. (f)CSNK1A1siRNA knockdown samples described inewere subjected to LC-MS/MS analysis for phospho-peptide mapping. The extracted-ion chromatogram peak area extracted from the LC-MS/MS data was used to calculate the relative abundance of the detected phospho-peptide in different conditions. Graph shows the quantitative loss of ~70–80%, of pS908, pS910, pS935, pS955, pS973 and pS976 fromCSNK1A1compared with NTC siRNA samples for both WT (filled circles) and K1906M (open circles). Figure 3: CK1α directly phosphorylates LRRK2 in vitro and in vivo . ( a ) LRRK2 is a substrate of CK1α. CK1α phosphorylates LRRK2, in vitro , at S910, S935, S955 and S973 sites. Representative blots of three independent experiments. ( b ) Consensus sequence of CK1 phosphorylation. The S/Tp-X-X-S/T is the canonical phosphorylation motif [42] . Alternative phosphorylation motif of CK1 consists of an SLS motif followed by an acidic cluster in positions n +7 (underlined [43] ). Sequence analysis of LRRK2 shows that serines 910, 935 and other constitutively phosphorylated serines at 973/975/976 is a weak consensus site for canonical and noncanonical CK1α phosphorylation. Phosphorylated serines of LRRK2 are shown in red. ( c ) IC261, but not LRRK2-IN1, inhibited CK1α phosphorylation of LRRK2 in vitro . Concentrations of inhibitors used were 50 μM IC261 and 100 nM LRRK2-IN1. Results were consistent even when higher concentration of inhibitor, 100 μM IC261 and 1 μM LRRK2-IN1, was used ( Supplementary Fig. 4b ). Representative blots of three independent experiments. ( d ) Quantitation of blots in c . Graph shows mean±s.e.m. Statistical significance tested with two-way ANOVA with Bonferroni post hoc test (* P <0.05; ** P <0.01; n.s.=not significant). ( e ) LRRK2 is dephosphorylated at S910, S935, S955 and S973 upon knockdown with CSNK1A1 siRNA in a LRRK2-kinase-independent manner, as both WT and K1906M is dephosphorylated to the same extent. ( f ) CSNK1A1 siRNA knockdown samples described in e were subjected to LC-MS/MS analysis for phospho-peptide mapping. The extracted-ion chromatogram peak area extracted from the LC-MS/MS data was used to calculate the relative abundance of the detected phospho-peptide in different conditions. Graph shows the quantitative loss of ~70–80%, of pS908, pS910, pS935, pS955, pS973 and pS976 from CSNK1A1 compared with NTC siRNA samples for both WT (filled circles) and K1906M (open circles). Full size image It is possible that other kinases are involved in phosphorylating LRRK2 at S910/S935. From our screen, CK1α and WEE1 were two candidate kinases, which, upon knockdown, resulted in the loss of pS935. We therefore performed an in vitro kinase assay of WEE1 and LRRK2, as we did for CK1α. Our results show that WEE1 does not phosphorylate LRRK2 in vitro at S910/S935/S955/S973 ( Supplementary Fig. 5a ) despite confirming that the WEE1 used in these experiments was kinase-active ( Supplementary Fig. 5b ). Since CK1α is one of six isoforms within the casein kinase family, we also investigated whether the other isoforms can phosphorylate LRRK2 at the interrogated phosphosites. We performed in vitro kinase assays against LRRK2 for each human CK1 isoform (alpha, delta, epsilon, gamma 1, gamma 2 and gamma 3). Although phosphorylation at S910/S935/S955 was strongest for CK1α, we found that CK1δ/ε and CK1γ isoforms could moderately phosphorylate S955 and S935 in vitro , respectively ( Supplementary Fig. 5c,d ). We therefore asked whether the identification of CK1α from the initial siRNA screen and subsequent validation was related to targeting of other CK1 isoforms in HEK cells. siRNA against CK1α did not affect the expression of the other CK1 isoforms (δ, ε and γ1), implying that the loss of pS935 in cells was likely due to CK1α knockdown ( Supplementary Fig. 5e,f ). Collectively, these results support the hypothesis that CK1α is a direct kinase for LRRK2 at multiple constitutive phosphorylation sites in HEK cells, although in other tissues it is possible that other CK1 isoforms might contribute to LRRK2 phosphorylation. We also asked whether there were additional phosphorylation sites in LRRK2 that are phosphorylated by CK1α. Wild-type or kinase dead LRRK2 was purified from HEK293FT cells and shown to be dephosphorylated at S910, S935, S955 and S973 upon knockdown with CSNK1A1 siRNA in a LRRK2-kinase-independent manner using antibodies to these sites ( Fig. 3e ). Using mass spectrometry ( Fig. 3f ), we identified a total of six phospho-peptides responsive to CK1α knockdown, four that were consistent with the antibody results (pS910, pS935, pS955 and pS973) as well as two additional sites (pS908 and pS976). Quantitatively, there was a reduction in the relative abundance of all detected LRRK2 phospho-peptides, expressed as extracted-ion chromatogram peak area within ±0.01 Da of monoisotopic mass of each phospho-peptide ( Supplementary Fig. 6 ), from CSNK1A1 compared with non-targeting control (NTC) siRNA samples for both WT and K1906M ( Fig. 3f , Supplementary Table 1 ). There was ~75% reduction for the more abundant sites (pS908/S910/S935) and diminishment below the level of detection for the less phosphorylated sites (pS955/S973/S976) when CK1α is knocked down in WT and K1906M. Therefore, our results show that LRRK2 phosphorylation at all identified phosphorylation sites is dependent on CK1α in an intact cell system. LRRK2 GTP binding is regulated by CK1α and ARHGEF7 The above results provide tools to dissect out kinase activity of LRRK2 from its constitutive phosphorylation. Specifically, we reasoned that by contrasting the effects of LRRK2-IN1, which would trigger dephosphorylation of LRRK2 and inhibit its kinase activity, compared with IC261, which should leave LRRK2 kinase active but dephosphorylated, we could infer which properties were related to constitutive phosphorylation and which to acute kinase inhibition. Because of the multiple serines that are phosphorylated in the region between S908 and S976, we reasoned that inhibition of CK1α would provide a more reliable loss of all phosphorylation sites than mutagenesis to alanine of selective sites such as S910A/935A and would also allow for temporal control of phosphorylation of LRRK2. During validation of the effect of LRRK2-IN1 on LRRK2, we found that inhibition of kinase activity combined with loss of phosphorylation had differential effects on protein interaction of LRRK2. Specifically, and as widely reported, 14-3-3 binding was lost but Hsp90 binding was retained ( Supplementary Fig. 1b,c ). We therefore considered whether differential protein interactions might be relevant to any downstream effects of CK1α inhibition. Using co-immunoprecipitation, we found that CK1α and LRRK2 had a measureable, albeit weak interaction. The apparent strength of this interaction was diminished after treatment with LRRK2-IN1 or IC261 for WT and S910A/935A, but was only diminished with IC261, not LRRK2-IN1, for the kinase dead K1906M variant ( Fig. 4a,b ). These results show that CK1α binding to LRRK2 depends both on LRRK2 kinase activity and on phosphorylation at constitutive sites, supporting our contention that comparing the two inhibitors can yield novel insights into LRRK2 interactions. We therefore extended these studies to additional protein interactions. 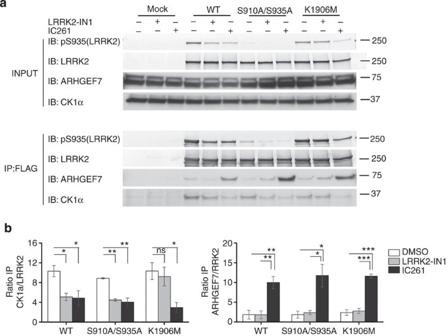Figure 4: LRRK2 differentially interacts with CK1α and ARHGEF7 upon loss of constitutive phosphorylation. (a) CK1α and ARHGEF7 are binding partners of LRRK2. When pS935 is lost, either due to 1 μM LRRK2-IN1 or 200 μM IC261 treatments, CK1α interaction with LRRK2 is diminished. Association of ARHGEF7 with LRRK2 (WT, S910A/S935A and K1906M) was increased upon IC261 treatment but no change in LRRK2–ARHGEF7 association occurred after LRRK2-IN1 treatment. Representative blots from three independent experiments. (b) Quantitation of blots ina. Graph shows mean±s.e.m. Statistical significance tested with one-way ANOVA with Tukey’spost hoctest comparing treatments within a group (*P<0.05; **P<0.01; ***P<0.001; n.s.=not significant). Figure 4: LRRK2 differentially interacts with CK1α and ARHGEF7 upon loss of constitutive phosphorylation. ( a ) CK1α and ARHGEF7 are binding partners of LRRK2. When pS935 is lost, either due to 1 μM LRRK2-IN1 or 200 μM IC261 treatments, CK1α interaction with LRRK2 is diminished. Association of ARHGEF7 with LRRK2 (WT, S910A/S935A and K1906M) was increased upon IC261 treatment but no change in LRRK2–ARHGEF7 association occurred after LRRK2-IN1 treatment. Representative blots from three independent experiments. ( b ) Quantitation of blots in a . Graph shows mean±s.e.m. Statistical significance tested with one-way ANOVA with Tukey’s post hoc test comparing treatments within a group (* P <0.05; ** P <0.01; *** P <0.001; n.s.=not significant). Full size image ARHGEF7 was reported to bind to the ROC domain of LRRK2 and suggested to induce LRRK2 autophosphorylation [24] . We first investigated whether the interaction of LRRK2 and ARHGEF7 was altered upon treatment with LRRK2-IN1 or IC261. Treatment with IC261 increased LRRK2 association with endogenous ARHGEF7 for WT, S910A/S935A and K1906M, accompanied by loss of constitutive phosphorylation ( Fig. 4b ). In contrast, LRRK2-IN1 did not cause a change in LRRK2–ARHGEF7 association. This suggests that interaction between LRRK2 and ARHGEF7 depends on both phosphorylation and kinase activity of LRRK2. Given that ARHGEF7 differentially interacts with LRRK2 after IC261 compared with LRRK2-IN1 treatments, we asked whether this differential interaction might alter GTP binding for the overall complex of LRRK2 with ARHGEF7 and potentially other GTPases (see Discussion). Treatment of cells with 1 μM LRRK2-IN1 increased GTP binding for all tested forms of LRRK2 except Y1699C and K1906M ( Fig. 5a,b ). In contrast, treatment with IC261 decreased GTP binding for all variants ( Fig. 5a,b ). These results show that dephosphorylation of LRRK2 when present as part of a complex with ARHGEF7, and possibly other GTPases, diminishes the apparent affinity of LRRK2 for GTP. 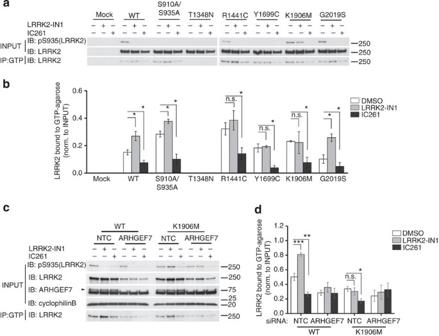Figure 5: Loss of constitutive phosphorylation alters ARHGEF7-mediated LRRK2 GTP binding. (a) GTP-binding assay for LRRK2 from transfected HEK293FT cells treated with 1 μM LRRK2-IN1 or 200 μM IC261 for 2 h. Kinase inhibition with LRRK2-IN1 increased LRRK2 GTP binding, whereas reduction of GTP binding was observed with IC261. The effect of IC261 was consistent for all variants, including K1906M. Representative blots from three independent experiments. (b) Quantitation of blots ina. GTP-bound LRRK2 normalized to amount of LRRK2 in input. Data are from three independent experiments (mean±s.e.m.). Statistical significance tested using unpairedt-test (treatment compared with DMSO control; *P<0.05; ns, not significant). (c) Alterations of LRRK2 GTP binding observed due to LRRK2-IN1 and IC261 treatments were abolished upon knockdown of ARHGEF7 using siRNA. Arrow shows ARHGEF7 protein in NTC samples but is not detected in ARHGEF7 siRNA samples. Representative blots from four independent experiments. (d) Quantitation of blots inc. Graph shows mean±s.e.m. Statistical significance tested with one-way ANOVA with Tukey’spost hoctest comparing treatments within a group (*P<0.05; **P<0.01; ***P<0.001; ns, not significant). Figure 5: Loss of constitutive phosphorylation alters ARHGEF7-mediated LRRK2 GTP binding. ( a ) GTP-binding assay for LRRK2 from transfected HEK293FT cells treated with 1 μM LRRK2-IN1 or 200 μM IC261 for 2 h. Kinase inhibition with LRRK2-IN1 increased LRRK2 GTP binding, whereas reduction of GTP binding was observed with IC261. The effect of IC261 was consistent for all variants, including K1906M. Representative blots from three independent experiments. ( b ) Quantitation of blots in a . GTP-bound LRRK2 normalized to amount of LRRK2 in input. Data are from three independent experiments (mean±s.e.m.). Statistical significance tested using unpaired t -test (treatment compared with DMSO control; * P <0.05; ns, not significant). ( c ) Alterations of LRRK2 GTP binding observed due to LRRK2-IN1 and IC261 treatments were abolished upon knockdown of ARHGEF7 using siRNA. Arrow shows ARHGEF7 protein in NTC samples but is not detected in ARHGEF7 siRNA samples. Representative blots from four independent experiments. ( d ) Quantitation of blots in c . Graph shows mean±s.e.m. Statistical significance tested with one-way ANOVA with Tukey’s post hoc test comparing treatments within a group (* P <0.05; ** P <0.01; *** P <0.001; ns, not significant). Full size image To explore the mechanism(s) behind these observations, we considered several alternative models. CK1α knockdown with siRNA or inhibition with IC261 did not induce LRRK2 autophosphorylation at sites within the ROC domain, as we were unable to detect these events in cell lysates ( Supplementary Fig. 7a,b ). These results therefore do not support one possible model whereby LRRK2 phosphorylates itself to regulate GTP binding directly. We further noted that the alteration in GTP binding only occurred when the assay was carried out using cell lysates, and not with purified LRRK2 ( Supplementary Fig. 8a,b ), suggesting that the change in GTP binding is not due to an alteration in the intrinsic property of LRRK2 but rather a change in association with its binding partner(s). We therefore repeated the GTP-binding assay in cells with ARHGEF7 knockdown. The effects of LRRK2-IN1 and IC261 on GTP binding of either WT or kinase dead LRRK2 were abolished by siRNA against ARHGEF7 ( Fig. 5c,d ). These results show that the effects of LRRK2 dephosphorylation on GTP binding depends not on LRRK2 directly but on interacting protein(s), including ARHGEF7. Consistent with previously published work from ref. 24 , we found that LRRK2 could phosphorylate ARHGEF7 in vitro ( Supplementary Fig. 9 ), adding further complexity to the model of regulation of GTP binding via a LRRK2/ARHGEF7 complex. We therefore felt that it was important to establish whether dephosphorylation of LRRK2, and associated altered GTP binding, might have consequential effects on cellular phenotypes related to expression of LRRK2 and its binding partners. CK1α negatively regulates LRRK2 and TGN clustering ARHGEF7 has been shown to play a role in the Rac1-dependent actin polymerization on trans -Golgi network (TGN) [25] . We have recently demonstrated a functional link between LRRK2 and TGN46-positve Golgi clustering and clearance that further depends on the small GTPase Rab7L1 (ref. 18 ). Given the overlap in the role of LRRK2, Rab7L1 and ARHGEF7 at the TGN, we therefore investigated the effect of CK1α and ARHGEF7 on LRRK2 relocalization and Golgi clustering when co-expressed with Rab7L1. Our previous assays of TGN clustering were based on manual counting of TGN46-positive structures in cells [18] . In order to assure that the same phenotypes could be monitored in an unbiased manner, we developed an objective morphological assay for LRRK2/Rab7L1 relocalization to the TGN based on an automated microscopy platform (see Methods). We confirmed that this version of the assay worked as expected by demonstrating that LRRK2/TGN46 clustering was promoted by WT Rab7L1 but not by the Q67L Rab7L1 mutant that does not retain GTP (ref. 18 ) ( Fig. 6a,b ). Knockdown of Rab7L1 also diminished TGN46 localization, as expected ( Fig. 6b ). Furthermore, knockdown of ARHGEF7 also prevented clustering of TGN but knockdown of CK1α increased the proportion of cells where LRRK2 and Rab7L1 were recruited to the TGN ( Fig. 6b ). These data show that constitutive phosphorylation of LRRK2 modulates its recruitment, in an ARHGEF7-dependent manner, to TGN46-positive Golgi organelles and suggest that CK1α has physiologically relevant effects on LRRK2 phenotypes. 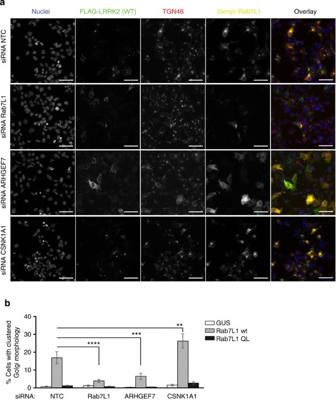Figure 6: CK1α negatively regulates ARHGEF7-mediated Rab7L1-dependent LRRK2 localization and Golgi clustering. (a) 293FT cells were co-expressed with FLAG-tagged LRRK2 and either with myc-tagged GUS (negative control for transfection), Rab7L1 WT or Q67L (loss of function variant), and also transfected with siRNA againstRab7L1,ARHGEF7orCSNK1A1. Cells were stained for FLAG (green), TGN46 (red), myc (yellow) and nucleus (blue). The assay was set up in a 96-well plate format and the Golgi phenotype was imaged on a Cellomics VTI arrayscan. An automated counting of cells with LRRK2/TGN46-positve Golgi clustering was performed using the spot detector bioapplication of the Cellomics software to avoid operator bias. Scale bar shown is 50 μm. (b) Quantitation of proportion of cells with Golgi clustering phenotype shown ina. Data are from three independent experiments with six wells per condition and 1,000 cells were counted per well. Graph shows mean±s.e.m. Statistical significance tested with two-way ANOVA with Tukey’spost hoctest comparing test siRNA to NTC within a group (**P<0.01; ***P<0.001; ****P<0.0001). Figure 6: CK1α negatively regulates ARHGEF7-mediated Rab7L1-dependent LRRK2 localization and Golgi clustering. ( a ) 293FT cells were co-expressed with FLAG-tagged LRRK2 and either with myc-tagged GUS (negative control for transfection), Rab7L1 WT or Q67L (loss of function variant), and also transfected with siRNA against Rab7L1 , ARHGEF7 or CSNK1A1 . Cells were stained for FLAG (green), TGN46 (red), myc (yellow) and nucleus (blue). The assay was set up in a 96-well plate format and the Golgi phenotype was imaged on a Cellomics VTI arrayscan. An automated counting of cells with LRRK2/TGN46-positve Golgi clustering was performed using the spot detector bioapplication of the Cellomics software to avoid operator bias. Scale bar shown is 50 μm. ( b ) Quantitation of proportion of cells with Golgi clustering phenotype shown in a . Data are from three independent experiments with six wells per condition and 1,000 cells were counted per well. Graph shows mean±s.e.m. Statistical significance tested with two-way ANOVA with Tukey’s post hoc test comparing test siRNA to NTC within a group (** P <0.01; *** P <0.001; **** P <0.0001). Full size image Understanding the impact of constitutive phosphorylation on LRRK2’s biochemical and cellular phenotype may be important for understanding the disease process as pathogenic PD mutations are associated with decrease in phosphorylation at these sites [9] , [13] , [17] . Here we provide evidence using multiple techniques that CK1α is an upstream kinase responsible for LRRK2 phosphorylation at a series of constitutive phosphorylation sites. The identification of CK1α as an immediate kinase for LRRK2 is based on four major pieces of evidence: (1) an unbiased siRNA screen; (2) validation of that screen using individual and pooled siRNAs; (3) pharmacological confirmation using CK1 versus CK2 inhibitors and (4) reconstitution of the effects in vitro using purified proteins. We used both antibody and mass spectrometry-based approaches to support these conclusions, with similar results. The effects of CK1 inhibitors are not limited to dividing cells or to overexpressed proteins as the same effect can be replicated with endogenous LRRK2 in neurons and in acute adult brain slices. Interestingly, CK1 inhibitors diminish phosphorylation of both kinase-active and kinase dead versions of LRRK2. This demonstrates for the first time that the constitutive phosphorylation of K1906M can be manipulated and contrasts with the effects of loss of phosphorylation of LRRK2 that results from LRRK2 kinase inhibition, which presumably proceeds by a feedback mechanism. Furthermore, this provides tools whereby kinase activity of LRRK2 and regulation by other kinases can be dissociated, which may be useful for developing novel therapeutic approaches. Inhibition of LRRK2 kinase activity promotes an increase in the binding of LRRK2 complexes to GTP for all kinase-active LRRK2 variants except for Y1699C. Interestingly, the opposite was observed for IC261, where all variants including K1906M had decreased GTP binding. The relationship between kinase activity of LRRK2 and GTP binding and hydrolysis by the ROC–COR bidomain has been controversial. Early models suggested that GTP binding in the ROC–COR domain would stimulate kinase activity, analogous to the regulation of Raf kinases by Ras GTPases. However, several pieces of data challenge this simple model, including that, while adding GTP to cell lysates will modestly stimulate kinase activity of LRRK2, the same addition to purified LRRK2 has no effect [26] , [27] . Characterization of autophosphorylation of LRRK2 identified sites within the ROC domain as targets of LRRK2 kinase activity. However, the evidence that such events occur in cells (as distinct from in vitro ) has been modest, making the model of GTP regulation by kinase activity also uncertain. On the basis of the current data, we propose that the relationship between LRRK2 kinase and GTP-binding domains depends on phosphorylation at constitutive sites. Furthermore, we show that these effects are not due to direct action on LRRK2 but are dependent on regulated interaction with at least one other protein, ARHGEF7. It has been suggested previously [24] that association of ARHGEF7 and LRRK2 could lead to activation of LRRK2 GTPase activity, LRRK2 auto- and substrate phosphorylation and that ARHGEF7 might act as a guanine nucleotide exchange factor (GEF) for LRRK2 itself. When constitutive phosphorylation is lost upon treatment with IC261, LRRK2 showed enhanced associated with ARHGEF7, but this was not accompanied by an activation of autophosphorylation of LRRK2. We were able to reproduce the reported observation [24] that LRRK2 can phosphorylate ARHGEF7 in vitro , suggesting that there are signalling events within a putative LRRK2/ARHGEF7 complex that would be of interest to characterize further in future studies. We have not addressed whether ARHGEF7 acts as a classical GEF for LRRK2; however, we have shown that endogenous ARHGEF7 is necessary to mediate the changes in LRRK2 GTP binding after treatment with IC261. LRRK2 has been shown to bind to several small GTPases (Rac1 (ref. 28 ), Cdc42 (ref. 24 ), Rab5b (ref. 29 ), Rab7 (refs 30 , 31 ), Rab7L1 (refs 18 , 19 )) and some of these small GTPases also associate with the same putative GAPs and GEFs reported for LRRK2 (RGS2 (ref. 32 , 33 ), ArfGAP1 (refs 34 , 35 ) and ARHGEF7 (refs 24 , 25 , 28 , 36 )). Thus, it is possible that the apparent affinity of LRRK2 for GTP could be influenced by a combination of these GTP modulators. The exact stoichiometry and combination of proteins that make up a functional GTPase or kinase complex and how this regulation translates functionally in the cell is unknown and will require further investigation and a detailed dissection of the multivalent complex. Nonetheless, we provide some evidence that the relationship between LRRK2 and ARHGEF7 may involve LRRK2 phosphorylation by CK1α and Rab7L1 activity in the maintenance of the TGN. Rab7L1 and ARHGEF7 are both known to be involved in membrane trafficking of the Golgi, endoplasmic reticulum and endosomes [18] , [19] , [37] , [38] , [39] . We showed that. when ARHGEF7 is knocked down by siRNA, TGN clustering as we have recently reported [18] is abolished, implying that ARHGEF7 is required for Rab7L1-mediated recruitment of LRRK2 to the TGN. Collectively, our data put CK1α and ARHGEF7 in the interactome network of Rab7L1, GAK and BAG5 (ref. 18 ) and support the previously suggested role for LRRK2 in TGN clustering and clearance. Furthermore, we now suggest that regulation of LRRK2 phosphorylation status may be a key activating step in this pathway ( Supplementary Fig. 10 ). In summary, we provide evidence that CK1α is a physiological kinase regulator of LRRK2 including in the brain. Our overall interpretation is that kinase regulation of LRRK2 is an important event mediated by CK1α. We present in this study a novel entry point to regulate LRRK2 phosphorylation and the downstream functional links pertaining to maintenance of the TGN. Future studies should be directed towards understanding the pathogenic effects of mutations in LRRK2 within this context. We note that mutations in LRRK2 associated with PD have either enhanced kinase activity or lower basal phosphorylation. We speculate that dephosphorylation might be an important initial activation event for LRRK2 and that its kinase activity is then important for later regulation of its protein complex, potentially including ARHGEF7. Future studies should also be directed at understanding whether this model has predictive value for pathogenic mechanisms in PD. Vectors and cell lines FLAG-tagged (3 × ) wild type was cloned in a pCHMWS plasmid (generous gift from Dr Jean-Marc Taymans, De Katholieke Universiteit van Leuven, Belgium) as previously described [15] . Mutations (T1348N, R1441C, Y1699C, K1906M and G2019S) were introduced using a QuikChange II XL Site-Directed Mutagenesis Kit (Stratagene). All plasmids were analysed with EcoRI and EcoRV restriction enzymes (Fermentas) and fully sequenced. HEK293FT cells (Invitrogen) were used for transient transfections, and for stable transfections we used with 293T stably expressing 3 × FLAG-LRRK2 (refs 16 , 20 ; generous gift from Dr Jean-Marc Taymans, KU, Leuven, Belgium). Chemicals and antibodies Chemicals and reagents used in this study were are as follows: LRRK2-IN1 (Tocris Bioscience Cat no. 4273), IC261 (Millipore Cat no. 400090), D4476 (Abcam Cat no. ab120220), TMCB (Millipore Cat no. 218718), GTP (Sigma Cat no.G8877), ATP (Sigma Cat no. A6419), protease inhibitor (Roche Cat no. 04693159001), phosphatase inhibitor (Thermo Scientific Cat no. 78427), GTP beads (Jena Bioscience Cat no. NU-412-10), EZview Red Protein G Affinity Gel (Sigma Cat no. E3403), EZview Red ANTI-FLAG M2 Affinity Gel (Sigma Cat no. F2426), 3 × Flag peptide (Sigma Cat no. F4799), 10 × TBS (KD Medical) and 4 × SDS sample buffer (Invitrogen Cat no. NP0008). Antibodies used for western blotting (WB) or immunocytochemistry (IC) were as follows: anti-pS935 (University of Dundee, Scotland; WB 1 μg ml −1 ), anti-pS935 (Abcam Cat no. ab133450; WB 1:1,000), anti-pS910 (Abcam Cat no. ab133449; WB 1:1,000), anti-pT1410 (Abcam Cat no. ab140107; WB 1:1,000), anti-pT1503 (Abcam Cat no. ab154423; WB 1:1,000), anti-LRRK2 (Epitomics Cat no. 3514-1; 1:5,000), anti-LRRK2 (Millipore Cat no. MABN40; WB 1:1,000), anti-CK1α (Santa Cruz Cat no. sc-6477; WB 1:2,000), anti-CK1δ (Santa Cruz Cat no. sc-55553; WB 1:1,000), anti-CK1ε (Santa Cruz Cat no. sc-6471; WB 1:1,000), anti-CK1γ1 (Santa Cruz Cat no. sc-18493; WB 1:1,000), anti-ARHGEF7 (Protein Tech Cat no. 14092-1-AP; WB 1:1,000), anti-Hsp90 (Cell Signalling Cat no. 4877; WB 1:2,000), anti-alpha-tubulin (Cell Signalling Cat no. 2125; WB 1:1,000), anti-14-3-3 (Santa Cruz Cat no. sc-629; WB 1:2,000), anti-cdc37 (Cell Signalling Cat no. 610576; WB 1:1,000), anti-TGN46 (AbD Serotec Cat no. AHP500G; IC 1:200), anti-actin (Sigma Cat no. A5441; WB 1:2,000), anti-FLAG (Sigma Cat no. F1804; WB 1:5,000, IC 1:500), anti-myc (Roche Cat no. 11667149001; WB 1:2,000, IC 1:500), horse radish peroxidase-conjugated secondary antibodies (Jackson Immunology; WB 1:5,000) and fluorescent-conjugated secondary antibodies (Jackson Immunology; WB 1:50,000, Life Technologies; IC 1:500). RNA interference screen and validation HEK 293T cells stably overexpressing FLAG-tagged LRRK2 WT were seeded in Opti-MEM with 10% fetal bovine serum (FBS) at a density of 5.0 × 10 3 cells per well in 96-well Poly-L-Lysine-coated plates (BD Bioscience). Cells were allowed to grow for 24 h at 37 °C and then transfected with pooled ON-TARGETplus siRNA from the human Protein Kinases libraries (Thermo), as well as NTC siRNA (Thermo), at a final concentration of 25 nM. Each 96-well plate of siRNA was used to transfect two replicate 96-well plates of cells. Transfection was carried out according to the manufacturer’s protocol, using DharmaFECT 1 transfection reagent (Thermo) and 50 μl Opti-MEM with 10% FBS was added to the wells after 24 h. Two hours before lysis, LRRK2-IN-1 was diluted in Opti-MEM with 10% FBS and added to the appropriate wells to a final concentration of 10 μM. At 48 h post transfection, cells were lysed in 1 × Cell lysis buffer (Cell Signaling Cat no. 9803), Complete-Mini protease inhibitor (Roche) and Halt phosphatase inhibitor (Thermo)) for 30 min at 4 °C with agitation. Lysates were clarified with a 96-well filter plate (PALL Acroprep, 1.2 μm Supor membrane) by centrifugation at 3,000 g for 10 min at 4 °C. For siRNA deconvolution and validation, the above protocol was followed except that individual siRNAs against CSNK1A1 were transfected at final concentrations of 6.25 nM, and pooled at a total concentration of 25 nM. Validation with small molecule inhibitors HEK 293T cells stably overexpressing FLAG-tagged LRRK2 WT and K1906M LRRK2 were seeded in Opti-MEM with 10% FBS at a density of 2.5 × 10 4 cells per well of 96-well Poly-L-Lysine-coated plates. Cells were allowed to grow for 24 h at 37 °C before inhibitor treatment. The CK1 inhibitors (D4476 and IC261), CK2 inhibitor (TMCB) and LRRK2-IN-1 were diluted from 1,000 × dimethyl sulphoxide (DMSO) stocks in Opti-MEM with 10% FBS and added to wells to the indicated final concentrations. Control wells were treated with corresponding dilutions of DMSO. After incubation at 37 °C for 2 h, cells were harvested as described above and subjected to western blot analysis. Primary cortical neuron cell cultivation and transfection C57BL/6J or Lrrk2 −/− newborn (P 0 ) pups were used for preparation of primary cortical neurons as was described previously [40] . Briefly, neuronal cells were dissociated by papain (Worthington), plated on poly-D-lysine-precoated coverslips (Neuvitro) in Basal Medium Eagle (Sigma-Aldrich) supplemented with B27, N2, glutaMAX-I (Invitrogen) and 0.45% glucose (Sigma-Aldrich). For endogenous LRRK2 experiments, neuronal culture was maintained and harvested at 14 DIV following treatments with inhibitors as described in figure legends. The Lrrk2 −/− mice, Camk2a-tTA/tetO-LRRK2 (ref. 41 ) were a generous gift from Dr Huaibin Cai (NIA/NIH). Animal procedures were conducted in compliance with the guidelines approved by the Institutional Animal Care and Use Committee of the National Institute of Child Health and Human Development. Ex vivo acute striatal slices Coronal brain slices (1 mm thick) containing the striatum were prepared from 4- to 9-week-old Lrrk2 +/+ or Lrrk2 −/− C57BL/6J mice [41] . Sections were recovered for at least 2 h at 32 °C in artificial cerebrospinal fluid containing 124 mM NaCl, 4.5 mM KCl, 2 mM CaCl 2 , 1 mM MgCl 2 , 26 mM NaHCO 3 , 1.2 mM NaH 2 PO 4 and 10 mM D-glucose, that was bubbled continuously with carbogen (95% O 2 /5% CO 2 ). After 2-h treatment with 1 μM LRRK2-IN1, 300 μM IC261 or DMSO; striata were dissected and lysed in buffer containing 10 mM Tris/HCl and 2% SDS, supplemented with protease inhibitors cocktail (Roche) and HALT phosphatase inhibitor cocktail (Thermo Scientific). Lysates were sonicated and subjected to western blot analysis. SDS–PAGE and western blot analysis Protein samples were prepared in SDS sample buffer and boiled for 95 °C for 10 min before electrophoresis on 4–20% TGX gels (Bio-Rad). Proteins were transferred to polyvinylidene difluoride membranes using the semi-dry Trans-Blot Turbo Transfer System (Bio-Rad). Membranes were blocked with 5% non-fat milk OmniBlok (American Bioanalytical Cat no. AB10109), probed with primary (1 h at room temperature or overnight at 4 °C) and secondary (1 h at room temperature) antibodies and detected with enhanced chemiluminescence (Pierce Cat no. 32132) using X-ray films (GE Cat no. 28-9068-35) or on a Storm 860 Molecular Imager. For fluorescent-based detection of western blots, instead of milk, Odyssey Blocking Buffer (Licor Cat no.927-40000) was used and detection of fluorescent signal was performed on an ODYSSEY CLx (Licor). Quantitation of western blots was performed using the ImageJ software (version 1.41, National Institutes of Health, USA) or Image Studio (Licor). Full-length images of main immunoblots are shown in Supplementary Figs 11-16 . Protein purification and immunoprecipitation For FLAG immunopurification of LRRK2 proteins for in vitro kinase assay, 293FT cells, either stably or transiently (24 h), expressing 3 × FLAG-LRRK2, were pretreated with DMSO or LRRK2-IN1 before harvesting and lysis (20 mM Tris-HCl, pH 7.5, 150 mM NaCl, 1% (v/v) Triton X-100, phosphatase and protease inhibitor) for 30 min at 4 °C. Lysate was precleared with EZview Red Protein G Affinity Gel for 30 min at 4 °C followed by immunopurification with EZview Red ANTI-FLAG M2 Affinity Gel for 1 h at 4 °C. Protein–gel complexes were washed six times with wash buffer (25 mM Tris-HCl, pH 7.5, 400 mM NaCl, 1% (v/v) Triton X-100) and twice with kinase buffer (25 mM Tris-HCl, pH 7.5, 2 mM dithiothreitol, phosphatase inhibitor, 0.02% (v/v) Triton X-100). LRRK2 was eluted with 150 μg ml −1 3 × Flag peptide in kinase buffer for 30 min at 4 °C. Protocol for LRRK2 immunopurification was adapted for co-immunoprecipitation with modification to the lysis buffer (1 × TBS, 1 mM EDTA, 10% (v/v) glycerol, 0.3% (v/v) Triton X-100, phosphatase and protease inhibitor), wash buffer (1 × TBS, 0.1% (v/v) Triton X-100) and elution buffer (150 μg ml −1 3 × Flag peptide, kinase buffer and 400 mM NaCl). GTP-binding assay 293FT cells were transfected with FLAG-LRRK2 24 h before treatment with DMSO, LRRK2-IN1 or IC261 for 2 h before lysis. Cells were lysed in lysis buffer G (100 mM Tris-Cl, pH7.5, 50 mM KCl, 5 mM MgCl 2 , 1 mM EDTA, 1 mM EDTA, 10% (v/v) glycerol, 0.3% (v/v) Triton X-100, phosphatase and protease inhibitor) for 30 min at 4 °C. Total protein (100 μg) for each lysate sample, made up to a final volume of 500 μl, was incubated with 30 μl of GTP beads for 2 h at 4 °C. LRRK2-bound-GTP beads were washed twice with cold lysis buffer G and eluted from beads with 10 mM GTP for 15 min at 4 °C. Eluted samples and input were subjected to SDS–PAGE and western blotted for LRRK2. In vitro kinase assay LRRK2 was immunopurified, from cells treated with DMSO or LRRK2-IN1, as described above. Phosphorylation of LRRK2 by CK1 (α, δ, ε, γ1, γ2 and γ3) or WEE1 was measured in vitro via western blot analysis by detecting changes in pS910 and pS935 signal. Equal amounts of immunopurified LRRK2 per experiment were incubated with 100 μM nonradioactive ATP, 100 ng recombinant active CK1 isoforms (Signal Chem Cat no. C64-10G, C65-10G, C66-10G, C68-11G, C68-10BG and C68-10CG) or WEE1 (Active Motif Cat no. 31201) and with or without DMSO, LRRK2-IN1 and IC261, in a final volume of 20 μl in cold kinase buffer. To initiate reaction, the LRRK2-CK1 or WEE1 mix was incubated at 30 °C for 30 min, with continuous shaking. Reaction was terminated by adding SDS Sample buffer to a final 1 × concentration and boiled at 95 °C for 10 min. Samples were subjected to SDS–PAGE and western blot analysis as described above. Quantitative mass spectrometry phospho-peptide mapping LRRK2 was immunopurified from cells transfected with pooled NTC or CK1α siRNA at 25 nM for 48 h, as described above. Approximately 1.5 μg per purified LRRK2 protein sample was subjected to MS/MS for quantitative phospho-peptide mapping. Briefly, half of each sample was digested with chymotrypsin, and the other half was digested with trypsin. Liquid chromatography electrospray ionization tandem mass spectrometry (LC/MS/MS) experiments were performed using the digests. The LC/MS/MS data were searched against the NCBI Human database. Modifications included in the search are as follows: phosphorylation (Serine, Threonine, Tyrosine (STY)), Oxidation (M) and Carbamidomethyl (C). A decoy searching was also performed. The false discovery rate of the searches is less than 1%. Automated cellomic assay for LRRK2 and TGN46 HEK 293FT cells were seeded at 1 × 10 4 cells per well in a 96-well Matrigel-coated plate. Cells were transfected by reverse transfection with pooled ON-TARGETplus siRNA against ARHGEF7, CSNK1A1 or NTC (Thermo) at a final concentration of 25 nM. Transfection was carried out according to the manufacturer’s protocol, using DharmaFECT 1 transfection reagent (Thermo). Twenty-four hours after siRNA transfection, cells were further transfected with 3 × FLAG-LRRK2 and 2 × myc-GUS or 2 × myc-Rab7L1 WT or 2 × myc-Rab7L1 Q67L mutant plasmids using Lipofectamine-2000 (Life Technologies) reagent. Forty-eight hours after siRNA transfection and twenty-four hours after plasmid transfection cells were fixed with 4% paraformaldehyde containing 1 μg ml −1 Hoechst and stained for endogenous TGN46 (AbD Serotec), FLAG (Sigma) and myc (Roche) antibodies. Plates were imaged at × 20 objective on high-throughput Cellomics VTI arrayScanner and analysed using Spot Detector bioapplication for % of cells with LRRK2 and TGN46-positive spots from total number of LRRK2-transfected cells. Three independent experiments were performed with six wells per sample with the minimum of 1,000 cells per well. siRNAs samples for Rab7L1, ARHGEF7 or CK1α were compared with NTC within families (GUS, Rab7L1 WT or Rab7L1 Q67L) by two-way analysis of variance (ANOVA), Tukey’s multiple comparison test. Bioinformatics and statistical analyses For the siRNA screen for LRRK2 phosphorylation, we measured the ratio of S935 phosphorylated to total LRRK2 for each siRNA, with duplicate wells per siRNA. These values were initially normalized to the same ratio measured for recombinant LRRK2 on the same gel, and then adjusted for plate effects and transformed to a Z -based score representing deviation of this sample from the mean of the population (after adjustment) measured in s.d.’s. Adjusted Z -scores were then used to plot individual features for each replicate for each siRNA and candidate kinases were identified as those having Z below −3 for both replicates. When comparing the effects of LRRK2-IN1 or IC261 against DMSO treatment for each construct, we used unpaired Student’s t -test for two group comparisons or one-way ANOVA was used with Tukey’s post hoc test where there were more than two groups. In experiments where different LRRK2 constructs were used in the absence and presence of inhibitors, we used two-way ANOVA with mutant and treatment as factors, with Bonferroni post hoc test to compare the effects of LRRK2-IN1 or IC261 against DMSO treatment for each construct. How to cite this article: Chia, R. et al. Phosphorylation of LRRK2 by casein kinase 1α regulates trans -Golgi clustering via differential interaction with ARHGEF7. Nat. Commun. 5:5827 doi: 10.1038/ncomms6827 (2014).